The ghost of nestedness in ecological networks Ecologists are fascinated by the prevalence of nestedness in biogeographic and community data, where it is thought to promote biodiversity in mutualistic systems. Traditionally, nestedness has been treated in a binary sense: species and their interactions are either present or absent, neglecting information on abundances and interaction frequencies. Extending nestedness to quantitative data facilitates the study of species preferences, and we propose a new detection method that follows from a basic property of bipartite networks: large dominant eigenvalues are associated with highly nested configurations. We show that complex ecological networks are binary nested, but quantitative preferences are non-nested, indicating limited consumer overlap of favoured resources. The spectral graph approach provides a formal link to local dynamical stability analysis, where we demonstrate that nested mutualistic structures are minimally stable. We conclude that, within the binary constraint of interaction plausibility, species preferences are partitioned to avoid competition, thereby benefiting system-wide resource allocation. Nestedness has been studied in a wide range of ecological systems. The concept was first proposed in the early twentieth century but only became popular among ecologists with its application to the biogeographic pattern of species occurrence in islands and other fragmented landscapes [1] , [2] . More recently, nestedness in species interaction networks has received significant attention [3] , [4] , [5] , [6] , [7] , where it has been suggested that a nested pattern of interactions leads to greater biodiversity in mutualistic systems such as plant–pollinator networks [8] , [9] . In a nested bipartite network or graph, interactions are organized such that specialists (for example, pollinators that visit few plants) interact with subsets of the species with whom generalists (for example, pollinators that visit many plants) interact. A nested structure corresponds to a systematic arrangement of non-zero entries in the binary matrix used to represent a network, and existing detection methods are based on distinguishing the nested pattern from other possible arrangements of matrix elements [10] , [11] . However, these methods are often computationally expensive for large matrices and are not applicable to quantitative networks (binary metrics extended to work with quantitative data, such as WNODF [12] , do not make full use of the available quantitative information). Quantitative networks contain the number or frequency of pairwise interactions between species, and we show how empirical data can be rescaled to permit investigation of feeding or visitation preferences in addition to the basic presence–absence structure. If preferences are quantitatively nested, then the most generalist resources are preferred by all consumers—most strongly by generalist consumers, closely followed by specialist consumers—and specialist resources are neglected. We formally extend the definition of nestedness to include quantitative networks and propose a new and robust detection method based on the eigenvalue spectrum of a graph’s adjacency matrix. The spectral properties of perfectly nested graphs were first discussed in the mathematical literature, where they are known as double-nested graphs (DNGs) [13] or chain graphs [14] , and we show that large dominant eigenvalues are associated with highly nested structures (for both binary and quantitative matrices). A spectral method is advantageous because the eigenvalues of a matrix can be computed extremely quickly—even for large matrices—and results are invariant to matrix permutation [15] . Of 52 bipartite ecological networks from the literature, including plant–pollinator, parasitoid–host, and seed dispersal types, 51 (98%) were binary nested; however, only 3 (6%) had preference structures that were quantitatively nested. These results agree with our analysis of the dynamical (local) stability of nested graphs, where we demonstrate that perfectly nested configurations are minimally stable. Within the restriction of interaction plausibility—whether an interaction is forbidden or not, and identifiable with a binary structure [16] —species preferences are partitioned to avoid competition. Thus, ecological systems are organized such that niches are exploited and the efficient use of available resources is promoted. Nestedness and bipartite graphs Before explicitly considering ecological systems and empirical data, we begin by formally defining nestedness for both binary and quantitative bipartite networks, and present a general detection method that follows naturally from the matrix properties of nested graphs. A bipartite network or graph contains S nodes (species) that can be partitioned into two disjoint sets, A (animals in pollination networks) and P (plants), such that each of the E undirected edges (an animal–plant interaction) connects a node in the set A with another in the set P . For the binary case, the adjacency matrix is a square matrix in which if i and j are connected and is 0 otherwise; for quantitative networks can take positive non-zero values other than 1. The set of eigenvalues is an invariant property of a matrix (they do not change if rows and columns are permuted). Because is a symmetric matrix, all of its eigenvalues are real, and because the graph is bipartite, the eigenvalues are distributed symmetrically about 0. The largest eigenvalue of , the dominant eigenvalue, is known as its spectral radius , and for binary matrices its value is bounded from above by ( [13] , [15] ). Since matrix is symmetric and the graph bipartite, we need draw only the | P | × | A | incidence matrix (for example, Fig. 1 ). Nestedness can be defined as a property of the matrix . If is a perfectly nested binary matrix then there exists a permutation of rows and columns such that the set of edges in each row i contains the edges in row i +1, while the set of edges in each column j contains those in column j +1. More formally, the rows and columns of can be sorted (with ∀ j and ∀ i ) such that . This definition of perfect nestedness extends to quantitative as well as binary matrices. Matrices A , C , D , I , K and N in Fig. 1 are perfectly nested, as is matrix C in Fig. 2 , while the others are not. An example of perfect binary nestedness and the corresponding DNG notation used in graph theory is given in Supplementary Fig. S1 . 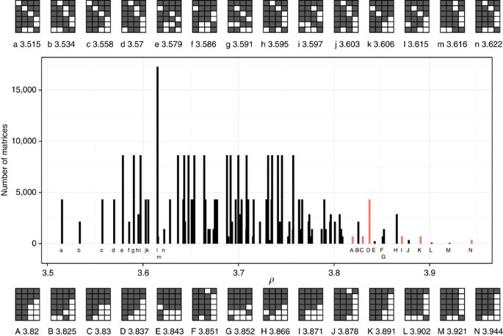Figure 1: Binary nestedness and eigenvalues. Spectral radius (ρ, largest eigenvalue) distribution for all connected graphs with |P|=6, |A|=4 and |E|=17. There are 346,104 possible incidence matrices with this parameter combination, and of these, 339,192 are connected (shown in the figure). Among the connected graphs, 7,560 are perfectly nested (coloured orange), and have higher spectral radii than most other matrices (all perfectly nested matrices are contained in the top 4.59% of the distribution). The maximum spectral radius is found for matrixN, and all matrices with spectral radius greater than that of matrixAare either perfectly nested or very close to being perfectly nested (bottom series): matricesB,E,F,G,H,J,LandMwould become perfectly nested if we were to move just one edge. Matrices with the lowest spectral radii depart most severely from perfect nestedness (top series). Figure 1: Binary nestedness and eigenvalues. Spectral radius ( ρ , largest eigenvalue) distribution for all connected graphs with | P |=6, | A |=4 and | E |=17. There are 346,104 possible incidence matrices with this parameter combination, and of these, 339,192 are connected (shown in the figure). Among the connected graphs, 7,560 are perfectly nested (coloured orange), and have higher spectral radii than most other matrices (all perfectly nested matrices are contained in the top 4.59% of the distribution). The maximum spectral radius is found for matrix N , and all matrices with spectral radius greater than that of matrix A are either perfectly nested or very close to being perfectly nested (bottom series): matrices B , E , F , G , H , J , L and M would become perfectly nested if we were to move just one edge. Matrices with the lowest spectral radii depart most severely from perfect nestedness (top series). 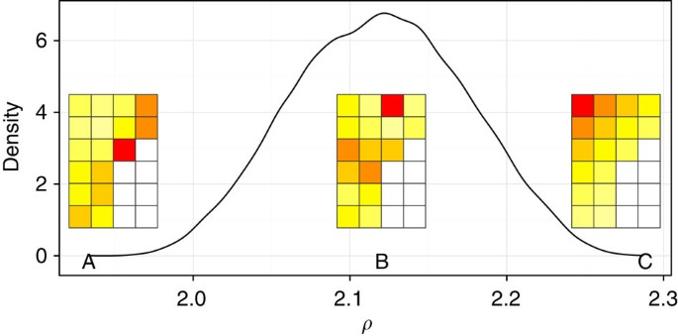Figure 2: Quantitative nestedness and eigenvalues. Spectral radius (ρ, largest eigenvalue) distribution for a perfectly nested binary structure (matrixAfromFig. 1) with randomized quantitative overlay. A single set of |E|=17 coefficient values are shuffled within the binary structure 10,000 times, and each time the spectral radius is computed. High spectral radius is associated with a highly nested quantitative configuration (for example, matrixC, where darker colours indicate higher relative element values), medium spectral radius with a non-specific quantitative configuration (for example, matrixB) and low spectral radius with an anti-nested quantitative configuration (for example, matrixA). Thus, the positive relationship between spectral radius and nestedness found for binary matrices extends to quantitative matrices. Full size image Figure 2: Quantitative nestedness and eigenvalues. Spectral radius ( ρ , largest eigenvalue) distribution for a perfectly nested binary structure (matrix A from Fig. 1 ) with randomized quantitative overlay. A single set of | E |=17 coefficient values are shuffled within the binary structure 10,000 times, and each time the spectral radius is computed. High spectral radius is associated with a highly nested quantitative configuration (for example, matrix C , where darker colours indicate higher relative element values), medium spectral radius with a non-specific quantitative configuration (for example, matrix B ) and low spectral radius with an anti-nested quantitative configuration (for example, matrix A ). Thus, the positive relationship between spectral radius and nestedness found for binary matrices extends to quantitative matrices. Full size image In the mathematical literature regarding DNGs, Bell et al . [17] provide a theorem that states: among all the connected bipartite graphs with | S | nodes and | E | edges, the one yielding the largest spectral radius is a perfectly nested graph. It was subsequently proved that the same holds if the number of nodes in each set P and A are fixed [18] , rather than choosing among all possible sizes such that | P |+| A |=| S | as in the original theorem. We confirm numerically that among all the bipartite graphs with | P | plants, | A | animals and | E | edges, the configuration leading to the largest spectral radius is a perfectly nested graph, with all other perfectly nested graphs having spectral radii close to this maximum value ( Fig. 1 and Supplementary Figs S2–S4 ). This finding extends to quantitative matrices and quantitative nestedness ( Fig. 2 ). The right tail of the spectral radius distribution contains either perfectly nested graphs—of which there can be many configurations (see Supplementary Methods )—or graphs that are very close to being perfectly nested, while the left tail contains graphs that are far from being perfectly nested. The spectral radius therefore represents a natural scale for nestedness, with larger obtained for more nested matrices with the same size and number of edges, and we have developed a set of statistical tests to determine the significance of nestedness for matrices that are not necessarily perfectly nested (see Methods and Supplementary Fig. S5 ). Matrices that are significantly non-nested in their binary form can become significantly nested when a sufficiently strong nested quantitative pattern is overlaid. This suggests that the quantitative structure of a network can dominate its underlying binary pattern ( Supplementary Fig. S6 ). The eigenvector associated with the spectral radius, besides being of interest in its own right [19] , provides a natural way of ordering nodes that best illustrates matrix nestedness. This follows from the standard eigenvalue equation : Because any eigenvector multiplied by the original adjacency matrix yields a vector parallel to the original adjacency matrix, the spectral radius (dominant eigenvalue) represents a scale factor λ for the dominant eigenvector. Conversely, if the spectral radius is understood to be a measure of nestedness, then the entries of the dominant eigenvector (of size the number of species) provide a way of ordering the species with respect to nestedness. Nestedness and ecological networks We now turn our attention to the specific case of ecological systems. In general, interactions among species can be described by a set of dynamical equations: , where x i is the density of a given species i , f ( x i ) describes the effect of its density on population growth and is the contribution to growth from interactions with other species in the system [20] , [21] , [22] . We can divide the interaction term between two species, , into two parts: the frequency of interactions γ i , j x i x j , and the effect of each interaction , and so . Typically, takes the form of a functional response that captures the effect of an interaction between i and all of its partners (for example, Holling’s Type II [23] ). For each pair of species, x i x j is a mass action term, and γ i , j indicates the relative frequency or probability of interaction compared to mass action. Under the mass action hypothesis, the basic affinity between two species—the expected magnitude of encounters—is directly proportional to the product of their densities, and factors such as the spatial layout of the environment, consumer search efficiency or handling time are not accounted for. These additional factors are aggregated in γ i , j . For each plausible ( γ i , j ≠0) interaction, γ i , j can be thought of as a preference parameter: if γ i , j >1 then the interaction is more likely to occur than expected and is therefore favoured, γ i , j <1 indicates that the interaction is less favourable and γ i , j =1 is exactly the expectation based on mass action. When we record ecological data such as the number of pollinator–plant visits—data that can be organized in the form of a quantitative incidence matrix —we implicitly record . So in practice, empirical data must be adjusted for mass action ( x i x j ) to isolate species preference γ i , j . We are particularly interested in whether the pattern of nestedness observed in binary bipartite ecological networks [4] is maintained in the quantitative preference structure represented by the γ -matrix. In a nested quantitative network, generalist–generalist species interactions are strongest, followed by generalist–specialist interactions, whereas specialist–specialist interactions are much weaker (and may be absent altogether). Effective abundance Before applying the tests for nestedness to empirical data, we first remove the effect of mass action in order to isolate species preferences. As interaction data are rarely accompanied by independent measures of species density, we use a method based on solving overdetermined sets of equations [24] to infer effective species abundances from quantitative interaction networks. These effective abundances should not be interpreted as field-measurable equivalents; rather, they are best-fit abundances under the mass action hypothesis. In some regards their use is more appropriate than the use of raw abundance data because they incorporate confounding factors such as life-cycle turnover, partner co-occurrence overlap and unevenness in spatial distribution. To obtain effective abundances, recall that we can write empirical count data . If no interaction is recorded, and we set the estimate for species preference . For the remaining set of recorded counts with , we take logarithms and perform a linear regression. However, rather than regressing ‘ y ’ against ‘ x ’ as is commonly done, we do the opposite such that we infer the log-transformed effective abundances and from the log-transformed counts (see Supplementary Methods ). The preference γ -term then represents errors or residuals, and as log γ i , j ’s are minimized during regression the estimated ’s are constrained to be as close to 1 as possible. In this way, binary matrices can be seen as a special case in which interaction magnitude is completely explained by mass action, and, as required, preferences are scaled relative to mass action—based on the inferred effective abundances—with . This quantitative -matrix can be assessed for nested patterns. Binary and quantitative nestedness of empirical networks We tested 52 bipartite empirical networks for binary and quantitative nestedness ( Table 1 and Supplementary Table S1 ). For each network and test, we computed the probability p that a randomly constructed matrix , which preserves some of the properties of the empirical adjacency matrix , is associated with spectral radius (see Methods). All but one of the networks were binary nested (defined as having P <0.05), in agreement with earlier studies [4] . However, nestedness was not observed in species preferences: for the vast majority of networks, the quantitative structure of the -matrix was indistinguishable from random configurations, and in some cases, anti-nestedness (defined as having P >0.95) became apparent ( Table 1 , Fig. 3 ). The lack of nestedness in the dominant quantitative structure of empirical networks is consistent with our mathematical treatment of the local stability of nested structures. Although local stability analysis captures only one aspect of ecological system dynamics, its mathematical tractability provides a good starting point for assessing the dynamical consequences of network structure [25] . Table 1 Nestedness of ecological networks using quantitative null model (iv) (maintain binary structure and shuffle non-zero coefficients, see Methods). 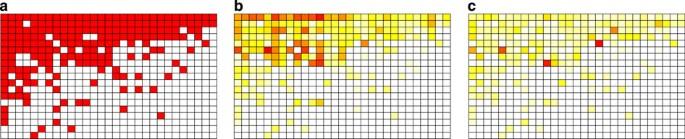Figure 3: Empirical nestedness. Three versions of a seed-dispersal mutualistic network with |P|=19, |A|=29 and |E|=211 (web 37 inSupplementary Table S1). In each incidence matrix, darker colours indicate higher relative element values. Applying tests for nestedness based on the spectral radius (see Methods) with 10,000 null model randomizations, we find: (a) the binary structure is nested,P<0.001 for the binary null model (i) and (ii); (b) the empirical count structure is quantitatively nested,P<0.05 for the quantitative null model (iv); and (c) the quantitative preference structure (the-matrix) is anti-nested,P>0.95 for the quantitative null model (iv). Therefore, within the restriction of interaction plausibility (matrixa), and after rescaling the raw data (matrixb) according to mass action, species preferences are found to be distributed in an anti-nested manner (matrixc). Full size table Figure 3: Empirical nestedness. Three versions of a seed-dispersal mutualistic network with | P |=19, | A |=29 and | E |=211 (web 37 in Supplementary Table S1 ). In each incidence matrix, darker colours indicate higher relative element values. Applying tests for nestedness based on the spectral radius (see Methods) with 10,000 null model randomizations, we find: ( a ) the binary structure is nested, P <0.001 for the binary null model (i) and (ii); ( b ) the empirical count structure is quantitatively nested, P <0.05 for the quantitative null model (iv); and ( c ) the quantitative preference structure (the -matrix) is anti-nested, P >0.95 for the quantitative null model (iv). Therefore, within the restriction of interaction plausibility (matrix a ), and after rescaling the raw data (matrix b ) according to mass action, species preferences are found to be distributed in an anti-nested manner (matrix c ). Full size image Local stability analysis Local stability analysis is concerned with how a dynamical system resting at equilibrium responds to perturbations. If an equilibrium point is stable, then the system returns to that point following small perturbations. For unstable equilibrium points, small perturbations will move the system away from the original resting state. Mathematically, the stability of an equilibrium point is completely defined by the sign of the real parts of the eigenvalues of the so-called community matrix M [25] , [26] , [27] (these eigenvalues are distinct from the adjacency matrix eigenvalues we have been considering so far). If all of the signs are negative then the equilibrium point is stable. Contemporary work has shown that nested mutualistic networks are less likely to be stable than their random counterparts [25] . We now demonstrate that a nested structure within M minimizes local stability. A community matrix can be written as the sum of a matrix with zeros on its diagonal, M ′, and a corresponding diagonal matrix, − D , that is, M = M ′− D . For very large systems, the spectral radius of M is , where is the average value of the diagonal [25] . Stability is therefore achieved whenever . Analogous to arranging coefficients in an adjacency or incidence matrix (as we did above), among all possible ways of arranging the coefficients of M ′ the configuration yielding the largest spectral radius is perfect nestedness (binary or quantitative). (Note that the community matrix is often considered non-symmetric, that is, the effect of an animal on a plant is often assumed to be different from that of the plant on the animal. However, the maximum spectral radius is obtained for symmetric matrices.) Hence, for a given diagonal and set of coefficients, nestedness of the community matrix minimizes local stability. This is seemingly at odds with the prevailing view that nestedness promotes the persistence of species in mutualistic systems [8] , [9] (although recent work has begun to question this proposition [28] ). As an approach to assessing system robustness, persistence encompasses local stability analysis—in many models of mutualism, local stability guarantees species persistence but locally unstable states may yet display persistence. Repeating precisely the analysis of Thébault and Fontaine [9] , we show that many dynamical models inadvertently build in trivial local stability and hence guarantee persistence: the diagonal elements of the community matrix are always large enough to compensate for the potential destabilizing effect of nestedness, thereby precluding nestedness—or, indeed, any other configuration of interactions—from having a significant contribution to local stability or persistence in such models (see Supplementary Methods and Supplementary Fig. S7 ). The claimed positive relationship between nestedness and persistence actually reflects a trivial positive relationship between connectance and persistence in obligate mutualistic systems—trivial because species without partners immediately go extinct (a feature not considered by Thébault and Fontaine [9] ), and species with initial densities close to zero will quickly go extinct unless they have sufficient (binary) mutualistic partners to ‘pull’ them to larger densities, after which they are guaranteed to persist [29] . Traditionally, nestedness has been associated with the plausibility of interaction: if the length of a pollinator’s proboscis is sufficient to obtain nectar from plants with deep corolla tubes, then it can also obtain nectar from species with shallower tubes, otherwise its visitation partners are restricted—for a community with many pollinator species, each with a different proboscis length, a nested binary interaction pattern emerges. Quantitative data allow us to investigate whether pollinators interact with particular plants more or less frequently than would be expected through random encounter, and whether they do so in any systematic fashion. With a nested preference structure, almost all consumers disproportionately interact with a common subset of the most generalist resources, while ignoring more specialist resources. While we found empirical networks to be binary nested, after adjusting for uneven species abundances according to mass action, their quantitative preference structures were distinctly non-nested. The need to account for abundances has been highlighted using synthetic networks, where heterogeneous abundance distributions combined with random species associations was sufficient to produce significantly nested binary patterns, leading to the conclusion that complex trait-based models were not necessary to explain nestedness [30] . Our results extend this argument to quantitative networks: The vast majority of empirical networks analysed had quantitative preference structures indistinguishable from random graphs, meaning that no systematic process is required to promote or constrain observed levels of nestedness. The lack of quantitative nestedness also finds support from mathematical analysis, where we showed that nested configurations of mutualistic interactions are minimally stable from the perspective of local stability analysis. How other types of interaction—such as antagonistic or facilitative pairings [8] —formally combine with mutualism to determine the overall stability and persistence of a network requires further work. At the community level, compared to quantitatively nested preference structures, non-nested structures suggest that species preferences are partitioned to avoid competition. Species rarely forgo abundant and accessible resources; rather, less abundant resources are disproportionately favoured by different sets of consumers—niches naturally arise. It would be instructive to see whether this kind of niche partitioning is also apparent at the level of individuals within a single-species population [31] . Much like the solar spectrum of light can be used to infer the constituent elements of our sun, we used a spectral approach—spectrum derived from the Latin for ghost—to detect nestedness in complex ecological networks. And like a ghost, nestedness, which was strongly apparent in binary structures, disappeared when quantitative preference structures were analysed. As the size of ecological data grows, the advantages of a spectral approach will become more pronounced; in addition to the dominant eigenvalue and eigenvector of a network’s adjacency matrix, considered here, the relationship between other spectral properties and ecological phenomena warrants further investigation. Our findings suggest that nestedness may not be the preeminent structure we once thought it was, but spectral analysis may further elucidate which structural features influence the function of large complex ecological networks. Tests for nestedness based on the spectral radius We showed that perfectly nested binary and quantitative matrices are associated with large spectral radius. Already, we have a strong test for nestedness: compute the spectral radius of an empirical matrix, and, if it is greater than the smallest spectral radius of a corresponding perfectly nested matrix, then the empirical matrix is almost guaranteed to be nested. However, in general, empirical data are incompatible with perfect nestedness (in many ecological networks, no super-generalists interacting with all of the species in the other class are observed). Here we describe four statistical tests for (not necessarily perfect) nestedness that are more applicable to real-world data sets. For each test, we compute the probability p that a randomly constructed incidence matrix has spectral radius , where and are the adjacency matrices of and , respectively. For both binary and quantitative matrices, we define three null models for constructing : (i) preserve | P |, | A | and place | E | edges at random within the matrix; (ii) as in (i), but accept only connected matrices; and (iii) as in (ii), but conserve the degree distribution (the row and column sums of ). As measures of nestedness can be very sensitive to matrix size, fill and configuration [10] , [11] , we used null model implementations that preserve | P |, | A | and | E | (null models (i) and (ii)) and degree distribution (iii) exactly, and not just their expected values. For quantitative matrices only, we introduce a fourth null model: (iv) preserve | P |, | A | and | E |, and shuffle the coefficient values of but not their positions. That is, maintain the binary structure of the matrix (where the non-zero entries are located) but randomize which coefficient values occupy which non-zero positions. Using this null model, the P -value is to equal to 1 when all the coefficients have the same value (for example, a binary matrix). In all tests, for all but the smallest of networks, P <0.05 is a suitable general significance level for nestedness, with P >0.95 indicating anti-nestedness. We encourage the use of null model (ii) for determining the nestedness of the binary network structure due to some important limitations of null models (i) and (iii), and null model (iv) for determining the nestedness of species preferences because it is the only null model that isolates quantitative structure (see Supplementary Methods ). Condition for finding connected graphs Null models (ii) and (iii) require connected matrices. To ensure that there is a reasonable probability of finding randomized matrices that are connected, we calculate the percolation point for random bipartite graphs. A classical result for Erdös–Rényi random graphs is the percolation point of connected graphs. For n nodes with a probability of connection C =| E |/(| P |·| A |), graphs in which C >log( n )/ n are almost surely connected, while those in which C <log( n )/ n are almost surely disconnected (for the limit n →∞). Without loss of generality, we will assume | P | ⩾ | A |. Saltykov [32] showed that in bipartite graphs the number of isolated nodes (that is, those that are not part of the giant component) is Poisson distributed. Using this result, Blasiak and Durrett [33] provided the following extension: for a random bipartite graph with | P | rows, | A | columns and | E | edges, whenever | E |>| P | log(| P |+| A |), the graph is almost surely connected (again, for the limit n →∞). From this, one can see that the probability of finding a connected graph approaches 1 whenever the probability of connection C >| P | log(| P |+| A |)/(| P |·| A |)=log(| P |+| A |)/| A |. For matrices with C around this threshold, it can take a long time to find connected matrices through random sampling. How to cite this article: Staniczenko, P.P.A. et al . The ghost of nestedness in ecological networks. Nat. Commun. 4:1391 doi: 10.1038/ncomms2422 (2013).